Encapsulated liquid sorbents for carbon dioxide capture Drawbacks of current carbon dioxide capture methods include corrosivity, evaporative losses and fouling. Separating the capture solvent from infrastructure and effluent gases via microencapsulation provides possible solutions to these issues. Here we report carbon capture materials that may enable low-cost and energy-efficient capture of carbon dioxide from flue gas. Polymer microcapsules composed of liquid carbonate cores and highly permeable silicone shells are produced by microfluidic assembly. This motif couples the capacity and selectivity of liquid sorbents with high surface area to facilitate rapid and controlled carbon dioxide uptake and release over repeated cycles. While mass transport across the capsule shell is slightly lower relative to neat liquid sorbents, the surface area enhancement gained via encapsulation provides an order-of-magnitude increase in carbon dioxide absorption rates for a given sorbent mass. The microcapsules are stable under typical industrial operating conditions and may be used in supported packing and fluidized beds for large-scale carbon capture. Reducing carbon dioxide (CO 2 ) emissions from coal-fired power plants is highly desirable. However, current systems for capturing carbon from flue gas are plagued by high capital, energy and chemical costs [1] , [2] , [3] , [4] , limiting their deployment to date. The most established technique for capturing CO 2 brings flue gas in contact with an aqueous amine solution, typically monoethanolamine (MEA), which reacts with CO 2 to form carbamates [5] . While MEA has a fast absorption rate and high CO 2 carrying capacity, it also possesses several drawbacks that prohibit widespread use [6] . MEA is highly corrosive, yields toxic degradation products, and requires significant energy to remove CO 2 during sorbent regeneration [7] , [8] , [9] , [10] , [11] . To overcome these limitations, new sorbents are needed. Recently, solid sorbents with high surface areas and low CO 2 binding energies, such as zeolites [12] , metal-organic frameworks [13] , [14] , [15] , frustrated Lewis pairs [16] and nanoporous polymers [17] , have been introduced; however, they suffer from low CO 2 capacity in the presence of water (which is abundant in flue gas), poor stability over multiple absorption–desorption cycles and/or high cost of production [5] , [18] , [19] . Here, we establish a new class of sorbent materials that combines the advantages of liquid solvents (that is, high capacity, high selectivity and water tolerance) and solid sorbents (for example, high surface area and low volatility). Specifically, we create highly permeable, microencapsulated carbon sorbents (MECS; Fig. 1a ). During absorption, CO 2 diffuses through the thin capsule shells, then dissolves and reacts in the liquid sorbent core to form the desired product(s). During regeneration, the reaction is reversed upon heating to yield high-purity CO 2 , which can subsequently be compressed for storage or utilization. Our core-shell MECS motif overcomes a central challenge in membrane-based gas separations [20] , where permeability and selectivity are often competing parameters [21] , since microcapsule permeability and sorbent selectivity can be independently optimized. The materials systems must meet several criteria; sorbent cores of controlled composition and geometry must be encapsulated, their polymeric shells (membranes) must be sufficiently permeable to CO 2 , so that the absorption rate is dominated by the encapsulated sorbent system, the sorbent system must be capable of multiple CO 2 absorption–desorption cycles, and the mechanical integrity of these microcapsules must be retained during repeated cycling. After evaluating a broad range of candidate materials, we identify a silicone shell that is both photocurable and chemically compatible with the sorbent system, which is composed of either an aqueous potassium carbonate (K 2 CO 3 ) or sodium carbonate (Na 2 CO 3 ) solution (core fluid). Potassium carbonate has long been used for CO 2 capture from natural gas in the Benfield Process [22] . More recently, carbonate solutions are being explored as an alternative to MEA for large-scale CO 2 capture from power plants [23] , [24] , because they are abundant, environmentally benign, resist degradation and have low volatility. Upon solid precipitation, carbonate slurries can be regenerated at modest or high temperature (80–150 °C) to yield purified CO 2 , resulting in a more energy-efficient capture process compared with that of MEA. Importantly, the main drawbacks of carbonate sorbents, that is, their slow CO 2 absorption kinetics and difficulty of handling precipitated solids in a liquid system, are overcome through encapsulation. Although corrosive or highly viscous ionic solvents may be encapsulated via the MECS motif yielding other types of capture media, we focus on carbonate solutions for this first demonstration. 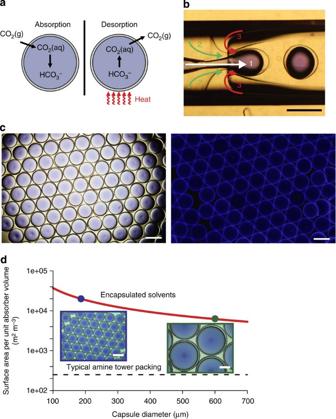Figure 1: Microcapsules for carbon capture. (a) Schematic illustration of the encapsulated liquid carbon capture process in which CO2(g) diffuses through a highly permeable silicone shell and is absorbed by a liquid carbonate core. The polymer microcapsules are then heated to release absorbed CO2for subsequent collection. (b) Image of the flow-focusing microfluidic capillary device used to produce the silicone microcapsules shown inc, where fluids 1, 2 and 3 correspond to the carbonate solution, ultraviolet-curable silicone and an outer aqueous solution, respectively. Scale bar is 250 μm in length. (c) Optical and fluorescent images of cured silicone microcapsules that possess uniform diameter (600±6 μm) and wall thickness (32±1 μm); scale bar, 1 mm. (d) Semi-log plot of available solvent surface as a function of microcapsule diameter. Insets: Optical images of silicone microcapsules assembled with varying diameters of 185 μm (left) and 600 μm (right). Dashed line denotes available surface area estimated for traditional CO2capture systems, in which monoethanolamine solution flows through a metal mesh-packed absorber tower. Scale bar, ~200 μm. Figure 1: Microcapsules for carbon capture. ( a ) Schematic illustration of the encapsulated liquid carbon capture process in which CO 2 (g) diffuses through a highly permeable silicone shell and is absorbed by a liquid carbonate core. The polymer microcapsules are then heated to release absorbed CO 2 for subsequent collection. ( b ) Image of the flow-focusing microfluidic capillary device used to produce the silicone microcapsules shown in c , where fluids 1, 2 and 3 correspond to the carbonate solution, ultraviolet-curable silicone and an outer aqueous solution, respectively. Scale bar is 250 μm in length. ( c ) Optical and fluorescent images of cured silicone microcapsules that possess uniform diameter (600±6 μm) and wall thickness (32±1 μm); scale bar, 1 mm. ( d ) Semi-log plot of available solvent surface as a function of microcapsule diameter. Insets: Optical images of silicone microcapsules assembled with varying diameters of 185 μm (left) and 600 μm (right). Dashed line denotes available surface area estimated for traditional CO 2 capture systems, in which monoethanolamine solution flows through a metal mesh-packed absorber tower. Scale bar, ~200 μm. Full size image Microcapsule design and fabrication Our MECS are produced using a double-capillary device [25] , which consists of nested glass capillaries fed by three fluids, whose flow rates are independently controlled shown in Fig. 1b . The inner fluid, that is, capsule core, is composed of an aqueous potassium or sodium carbonate solution with or without a pH indicator dye and catalyst for enhanced CO 2 absorption. The middle fluid (capsule shell) is a photopolymerizable silicone, and the outer (carrier) fluid is composed of an aqueous solution with stabilizer and surfactant. Double emulsion droplets are produced from the device at rates of 1–100 Hz ( Supplementary Movie 1 ), and subsequently cured by exposure to ultraviolet light to create microcapsules. Supplementary Fig. 1 shows a representative batch after collection and ultraviolet curing. Using this approach, we have prepared large quantities (>1 litre) of MECS filled with sorbent cores ranging in concentration from 3 to 30% by weight of potassium carbonate or sodium carbonate solutions. We chose fluid viscosities, flow rates and channel sizes that enable the fabrication of nearly monodisperse microcapsules with controlled outer diameters and shell wall thicknesses ranging from 100 to 600 μm and 10 to 50 μm, respectively. The permeability of CO 2 through the cured shell material was measured using a constant-volume, differential-pressure apparatus, in which pressure sensors on either side of the silicone membrane measure the rate of pressure change, or ‘leak-up’ rate, as the gas moves from the high pressure volume, through the membrane and into the low pressure volume (see Supplementary Methods ). The measured CO 2 permeability of the shell material is 3,260 barrer, which is quite high compared with most gas separation membranes [20] and comparable to values reported for other silicones [21] . Notably, this material exhibits no noticeable decrease in permeability after exposure to temperatures of up to 150 °C. The microcapsule geometries are highly uniform and can be readily adjusted by varying the fluid flow rates within the double-capillary device. Their initial and cured dimensions are determined using image analysis (see Supplementary Methods ). In Fig. 1c , optical and fluorescence microscopy images show a representative set of MECS that exhibit a highly uniform diameter (600±6 μm), wall thickness (31±1 μm) and centricity. Their physical dimensions can be systematically varied, as shown by the images of other representative batches with respective diameters of 185 and 600 μm produced using the same device under different operating conditions ( Fig. 1d , inset). Importantly, these geometries lead to a 1–2 orders of magnitude enhancement in sorbent surface area per volume of reactor relative to liquid in typical supported packing, shown in Fig. 1d (ref. 26 ). Although a simple packing of capsules in a tower would lead to a high pressure drop for gas flow, a supported packing that creates channels for flow or a fluidized bed would be suitable. CO 2 sorption and cycling To enable colorimetric observation of CO 2 absorption–desorption processes, we produced MECS containing a pH indicator dye, thymol blue, within their liquid sorbent cores. The unloaded potassium carbonate solution is blue and transforms to yellow when 90% of the maximum carbon uptake is achieved. This visible colour change serves as an effective colorimetric indicator of CO 2 saturation of the liquid carbonate sorbent, enabling qualitative monitoring of capsule loading and unloading. As a simple demonstration, we exposed MECS with liquid sorbent cores of 3 wt% K 2 CO 3 and thymol blue to air and to pure CO 2 . This K 2 CO 3 concentration is chosen to accommodate the solubility requirements of thymol blue, facilitating the colorimetric readout of capsule loading. Equilibrated in air, the microcapsules appear blue–violet. On exposure to the CO 2 atmosphere, the microcapsules quickly change to a deep, uniform yellow colour. After removing them from the CO 2 atmosphere, they return to their original blue–violet shade ( Fig. 2a–c ). This approach serves as a qualitative method of evaluating the absorption and desorption of CO 2 in ensembles of capsules during testing. On the basis of colorimetric analysis, their pH changes from ~10.2 to 9 (or lower) during CO 2 absorption and returns to its original value upon desorption (shown in Supplementary Fig. 2 ). To complement these data, we also use a manometric method to quantify CO 2 uptake. This method measures the pressure drop of CO 2 in a fixed volume as CO 2 is absorbed (see Methods). 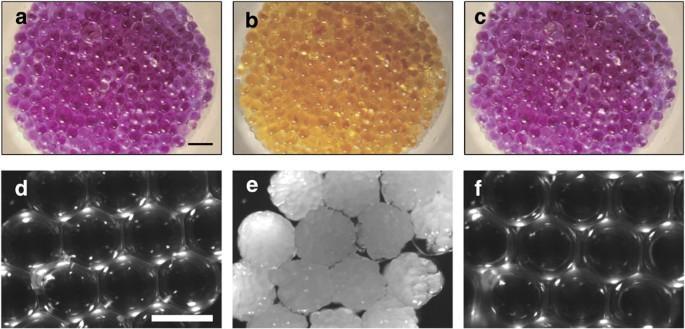Figure 2: CO2sorption and cycling. (a–c) Optical images of silicone microcapsules containing 3 wt% potassium carbonate dyed with thymol blue in air (a), after incubation in CO2gas (b) and then after regeneration in air (c). Scale bar, 1 mm. (d–f) Dark-field optical images of silicone microcapsules containing 30 wt% sodium carbonate in air (d), which were exposed to CO2gas until precipitation of bicarbonate from solution (e), and then regenerated by heating at 70 °C to release CO2gas and dissolve the precipitate (f). These microcapsules are mechanically robust, enabling repeated cycling of CO2capture and regeneration without degradation of the silicone shell walls. Scale bar, 500 μm. Figure 2: CO 2 sorption and cycling. ( a – c ) Optical images of silicone microcapsules containing 3 wt% potassium carbonate dyed with thymol blue in air ( a ), after incubation in CO 2 gas ( b ) and then after regeneration in air ( c ). Scale bar, 1 mm. ( d – f ) Dark-field optical images of silicone microcapsules containing 30 wt% sodium carbonate in air ( d ), which were exposed to CO 2 gas until precipitation of bicarbonate from solution ( e ), and then regenerated by heating at 70 °C to release CO 2 gas and dissolve the precipitate ( f ). These microcapsules are mechanically robust, enabling repeated cycling of CO 2 capture and regeneration without degradation of the silicone shell walls. Scale bar, 500 μm. Full size image Using this colorimetric method, we assessed the robustness of the microcapsule shells over multiple absorption–desorption cycles under realistic thermal cycling conditions. During cycling, polymer microcapsules are alternately exposed to CO 2 bubbled through water at 20 °C then heated to 40 °C and N 2 bubbled through water at 20 °C then heated to 100 °C in a custom apparatus. We monitored the colour changes and mechanical integrity via time-lapse photography over 80 cycles, and found that the colour change took place rapidly (<1 min) and the microcapsules not only remained intact throughout the entire testing period, but showed no apparent differences in their colorimetric response, indicating the shell material retains permeability ( Supplementary Fig. 3 ). We found that MECS are highly permeable to water as well as CO 2 , and reach osmotic equilibrium with their surroundings rapidly. Mechanical stability and crystallization We produced MECS containing 20–30 wt% Na 2 CO 3 and tested their mechanical integrity under highly alkaline, high ionic strength conditions during precipitate formation. The pH profiles of 20–30 wt% capsules are similar to the 3 wt% capsules as a function of fractional loading, and the kinetics are therefore similar, although their capacities are proportionally larger, akin to those targeted for industrial use. We find that the 30 wt% MECS can withstand a fourfold increase in their diameter without rupture by osmotically swelling in pure water ( Supplementary Fig. 4 ). Notably, this volumetric increase is far higher than that expected during their actual use as carbon capture media, where they will be held at osmotic equilibrium during storage. On exposure to a pure CO 2 atmosphere, we observe precipitate formation within their sorbent-filled cores as shown in Fig. 2d–f and Supplementary Movie 2 . These solid crystallites, confirmed by X-ray diffraction to be Nahcolite (NaHCO 3 ) ( Supplementary Fig. 5 ), enable enhanced carrying capacity and are thus beneficial for CO 2 capture. The solid precipitates repeatedly dissolve and reform upon cycling the microcapsules between a warm humid condition at 70 °C humidified to ~60% relative humidity (in which CO 2 and H 2 O is released) and CO 2 under ambient conditions ( Supplementary Fig. 6 ). The capacity of 30 wt% Na 2 CO 3 at equilibrium with flue gas with 0.1 bar CO 2 partial pressure allowing for the precipitation of NaHCO 3 (s) calculated to be 0.10 g CO 2 per gram solvent, as determined by Pitzer’s equations and GWB Software (see Supplementary Methods ) [27] , the same as MEA [28] . On the basis of previous analysis, the working capacity of sodium carbonate solution is slightly higher than MEA (7.1 versus 6.9% g per gram) [29] , [30] , but the values depend on process conditions. The shell material, whose thickness can be controlled, reduces the mass-basis working capacity of MECS. Compared with solid sorbents, sodium carbonate-filled MECS have capacities that are higher than hydrotalcites, similar to activated carbons, and lower than many zeolites (however, unlike most zeolites, their capacity is retained under humid conditions) [5] . The microcapsules remained mechanically stable even after cycling between air and pure CO 2 multiple times. Next, we analysed the amount of CO 2 released from these microcapsules during thermal desorption at 80 and 120 °C using pyrolysis–gas chromatography/mass spectrometry. These measurements revealed that only CO 2 and H 2 O evolve from the microcapsules at the two temperatures tested, indicating no degradation of the silicone material and release of a negligible fraction of other entrained gases. Accordingly, we calculate that in flue gas conditions, the quantity of dissolved O 2 and N 2 is about 10,000 times lower than that of absorbed CO 2 . N 2 and O 2 entrained in the shells and void spaces are expected to be similarly negligible. Overall, the selectivity of MECS for CO 2 is excellent compared with membranes and solid sorbents and comparable to liquid solvents. Like liquid solvents, MECS are expected to irreversibly bind SO x and NO x , but this has not yet been tested. The amount of CO 2 produced was ~0.90 mmol g −1 of capsules and 2.2 mmol g −1 of capsules at 80 and 120 °C, corresponding to 4.0 and 9.7% w/w, respectively. To explore the feasibility of MECS-based fluidized beds, we placed representative capsules containing 3 wt% potassium carbonate and thymol blue in a modified test tube. The capsules are first fluidized using N 2 gas, at a superficial velocity on the order of 1 m s −1 , which is in the range of velocities used in commercial fluidized beds [31] . The source gas is switched to pure CO 2 gas at equivalent velocity to the N 2 stream ( Supplementary Movie 3 ). We observed that the capsules change from blue to yellow in the presence of CO 2 . When the gas source is switched back to N 2 , their colour changes back to violet. This simple demonstration suggests that fluidized bed systems will provide an effective platform for carbon capture using MECS, since the capsules can survive rigorous agitation while functioning as effective carbon capture media. Enhancing capture kinetics To enhance their CO 2 capture kinetics, we produced MECS in which Zn-1,4,7,10-tetraazacyclododecane (‘cyclen’) is incorporated within the capsule cores (3 wt% potassium carbonate). Cyclen is a known mimic of the enzyme carbonic anhydrase and catalyses CO 2 absorption into aqueous solution [32] . We find that cyclen significantly increases the CO 2 absorption rates in carbonate solvents and remains stable at temperatures required for capsule regeneration. To monitor the effects of a catalysed liquid core, we placed MECS containing cyclen side-by-side with uncatalyzed MECS and exposed them to a CO 2 atmosphere. As shown in Fig. 3c–h and Supplementary Movie 4 , the catalysed microcapsules quickly absorbed CO 2 and reached saturation two to three times faster than those without catalyst. 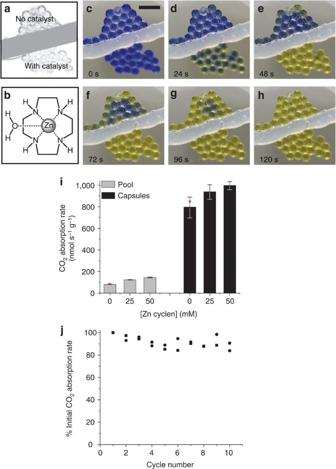Figure 3: Enhancing carbon capture kinetics via catalyst incorporation. (a–h) Optical images of silicone microcapsules filled with a 3 wt% potassium carbonate solution and Thymol Blue indicator in flowing CO2environment in the absence (top of panel) and presence (bottom of panel) of cyclen catalyst, schematically shown inaandb. The microcapsules exhibit a colorimetric change in pH (high to low) with CO2absorption along with an increased uptake rate in the presence of the catalyst (c–h). Scale bar, 1 mm. (i) Plot of CO2gas absorption rate for a liquid pool versus an encapsulated 3 wt% potassium carbonate solution with varying catalyst concentrations. Error bars correspond to the measured standard deviation for each system. Red stars denote the analytically predicted CO2absorption rate for the catalyst-free samples. (j) CO2absorption rate data for the microcapsules with 50 mM catalyst included over repeated absorption of carbon dioxide after steam regeneration cycles. The different symbols indicate two separate trials with the same conditions. Figure 3: Enhancing carbon capture kinetics via catalyst incorporation. ( a – h ) Optical images of silicone microcapsules filled with a 3 wt% potassium carbonate solution and Thymol Blue indicator in flowing CO 2 environment in the absence (top of panel) and presence (bottom of panel) of cyclen catalyst, schematically shown in a and b . The microcapsules exhibit a colorimetric change in pH (high to low) with CO 2 absorption along with an increased uptake rate in the presence of the catalyst ( c – h ). Scale bar, 1 mm. ( i ) Plot of CO 2 gas absorption rate for a liquid pool versus an encapsulated 3 wt% potassium carbonate solution with varying catalyst concentrations. Error bars correspond to the measured standard deviation for each system. Red stars denote the analytically predicted CO 2 absorption rate for the catalyst-free samples. ( j ) CO 2 absorption rate data for the microcapsules with 50 mM catalyst included over repeated absorption of carbon dioxide after steam regeneration cycles. The different symbols indicate two separate trials with the same conditions. Full size image The CO 2 absorption rates of MECS are measured quantitatively using a fixed-volume apparatus (see Methods). Control experiments are run with equivalent carbonate solutions in a pool of 1 mm depth, giving the same surface area-to-volume ratio as found for liquid solvents used in typical packed towers for CO 2 absorption [26] . The measured (mass normalized) CO 2 absorption rates for the MECS and control solutions (liquid pools) are shown in Fig. 3i . We observed a nearly 10-fold enhancement in absorption between these two configurations in the absence of cyclen. Further improvements (up to 12 × ) in CO 2 absorption rates are observed when comparing microcapsules with increasing catalyst concentrations to neat liquid sorbents of identical composition. These observations show that diffusion through the microcapsule shell is not a rate-limiting step, indicating that significant performance gains can be achieved by implementing the MECS motif. Maintaining activity over multiple absorption/desorption cycles is a necessary condition for their practical use. In addition to the 80-cycle colorimetric test described above, we directly measured MECS CO 2 absorption rates over 10 absorption–desorption cycles for two sets of microcapsules Fig. 3j . We found that the MECS retained at least 90% of their initial absorption rate during this testing process. We also compared the initial and final number of total moles of CO 2 absorbed per gram of capsules for the first and 10th absorption cycle, and found that capsules absorbed nearly equivalent (within 90% of initial equilibrium capacity) moles of CO 2 after 10 cycles. We compared the CO 2 absorption rate measurements of uncatalyzed capsules and solutions with theoretical predictions to gain understanding of the impact of our MECS motif. The absorption rate of pure carbonate solution (pool) can be estimated by [33] : where A is the interfacial area, is the partial pressure of CO 2 gas in the chamber and k solvent is the mass transfer coefficient of the solvent, which for carbonate solutions with low loading can be simplified to: where K H is the Henry’s constant for CO 2 , is the diffusivity of CO 2 in the solvent and k OH is the kinetic constant for reaction of CO 2 (aq) (equation (4) in Supplementary Methods ). We propose that the absorption rate of capsules can be estimated by: where P shell is the permeability of the shell material (in units of length 2 per time), and L is the thickness of the shell. Using the measured permeability along with reported values for other parameters, we calculate the absorption rates shown as stars in Fig. 3i . The measured rates for the liquid pool (control) and microcapsules are only slightly lower (~11–13%) than the calculated values; validating our approach of treating the microcapsules as a permeable membrane and solvent in series (more details are provided in Supplementary Methods ). Direct comparison between capsules and liquid pools at higher sodium carbonate concentrations, where crystallization occurs, is less straightforward, because Nahcolite at the air–solution interface inhibits diffusion of CO 2 into the unreacted solution. Silicone microcapsules filled with liquid carbonate sorbents exhibit an order-of-magnitude higher CO 2 absorption rate relative to neat sorbents of equivalent mass. The good agreement between predicted and measured mass transfer rates indicates that future development of encapsulated solvents can draw on extensive research on carbon capture liquids and gas separation membranes to inform both shell material and sorbent selection. We note that additional improvements in CO 2 capture rates can be achieved simply by optimizing the capsule geometry (for example, the smallest microcapsules produced have twofold higher surface area than those reported, Fig. 1d ). In addition, a broader range of sorbent and catalyst chemistries can be readily explored using this facile approach to achieve tailored functionality. These microcapsules are also well suited for use in supported packing or fluidized beds, as an important embodiment in their practical deployment. We have demonstrated a new class of hybrid liquid/solid materials that are highly permeable, mechanically robust, chemically stable and environmentally benign. Our encapsulation scheme enables the use of liquid sorbents with more favourable thermodynamics and lower environmental impact than MEA by improving mass transfer rates, containing precipitates, and isolating degradation products. A system based on concentrated sodium carbonate slurry can be run with less parasitic heating and evaporation of water than conventional amine systems and will not release toxic volatile organic compounds. Hence, microencapsulated carbon sorbents offer a promising approach for large-scale carbon capture from power plants that is both safer and more energy efficient than current alternatives. MECS fabrication Microcapsules are produced using a double-capillary device that consists of an outer square glass capillary, an inner circular capillary that has been flame polished and a final circular capillary that has been pulled to a fine tip. The pulled tip is drawn down using a laser tip puller to a final diameter of 30–40 μm. The two round capillaries are inserted into the square glass capillary. Epoxy is used to bond syringe tips to the capillaries and hermetically seal the device to the glass slide. Double emulsion droplets are produced by co-flowing three fluids in the device: (1) aqueous carbonate solution (inner fluid) for the carbon capture solvent, (2) a hydrophobic photopolymerizable silicone (middle fluid) (Semicosil 949UV, Wacker Chemie AG) for the shell material and (3) an aqueous carrier fluid with surfactant (outer fluid). After formation, the droplets exit the device and are collected in fluid and cured under ultraviolet light ( λ =365 nm). After curing, the polymerized microcapsules can be transferred and handled. After fabrication, microcapsules are stored in a potassium carbonate solution isotonic with the liquid sorbent cores to minimize osmotic swelling and rupture ( Supplementary Fig. 1 ). When the osmotic gradient is minimized, the microcapsules are stable for years with no apparent change in size or leakage. MECS characterization The introduction of a pH indicator dye, thymol blue, into the carbonate solvent before encapsulation enables visual confirmation that CO 2 is being absorbed by the encapsulated carbonate causing a pH swing. As the carbonate solution absorbs CO 2 , it reacts to form bicarbonate according to: while carbonate ions act as a buffer: Before CO 2 uptake, the dissolved carbon is present as carbonate in the initial ‘unloaded’ solution. By contrast, after CO 2 uptake, the carbon is present as bicarbonate leading to a reduction in the pH and a doubling of the initial carbon content in the fully ‘loaded’ solution. The calculated pH of the liquid sorbent core as a function of CO 2 absorption along with the corresponding thymol blue colour transition is provided in Supplementary Fig. 2 . A custom testing apparatus was built to controllably and rapidly cycle capsules between different gases and temperatures. In a single cycle, the microcapsules are first exposed to humid flowing nitrogen (N 2 ) gas at 40 °C to achieve temperature equilibration. Next, they are exposed to CO 2 gas at 40 °C for loading (CO 2 absorption). Finally they are exposed to N 2 gas at 100 °C for unloading (that is, CO 2 desorption). This was repeated for 80 cycles. For the fluidized bed test, capsules were first removed from the storage fluid, allowed to dry briefly in air, and then lightly powdered with potassium carbonate dust. The capsules were then loaded in a modified graduated cylinder with mesh blocking the inlets and outlets and connected to N 2 and CO 2 gas sources, flowing at a superficial velocity of 1.6 m s −1 for both gases. While N 2 was used to allow desorption at room temperature for this proof of concept testing, an industrial process is likely to regenerate at high temperature using CO 2 or a mixture of CO 2 and steam as the fluidization agent. Mass transfer measurements Absorption isotherms (equilibrium capacity) are typically reported for new solid sorbents. However, the vapour–liquid equilibria of carbonate solutions have been investigated previously [33] , [34] , and the MECS process is not expected to change the equivalent vapour–liquid equilibria of the encapsulated solvent. By contrast, absorption kinetics may be strongly affected by encapsulation. We therefore focused on measuring the rate of absorption at relevant CO 2 partial pressures. To measure CO 2 absorption kinetics, we suspended MECS on a steel mesh in a sealed, fixed-volume, temperature-controlled vacuum chamber equipped with a pressure gauge and a valve for the introduction of CO 2 ( Supplementary Fig. 7 ) [35] , [36] , [37] . Although gravimetric methods are typically used for solid sorbent investigations, that technique is complicated by water exchange in and out of the hybrid liquid–solid capsule system we investigate here. The mesh size was chosen to separate capsules from each other and maximize accessible surface area. The chamber was evacuated to the solution vapour pressure and a controlled quantity of CO 2 was introduced, followed by sealing the chamber and monitoring the total pressure over time. The water vapour pressure was assumed to remain constant and was subtracted from the total to give the CO 2 partial pressure. Typical raw data from this absorption measurement is shown in Supplementary Fig. 8 . As shown, both the absorption kinetics and the absorption capacity of the materials can be measured as the slope of the pressure versus time trace and the difference between the starting and final CO 2 partial pressures, respectively. For the control experiments, we created a small pool in the apparatus with a 1 mm depth, which is the average depth of solution on the packing in a typical packed tower for CO 2 capture. At low loading (high pH), stirring or flowing has little effect on the rate of CO 2 absorption of a carbonate solution since the rate is driven by reaction. Hence, the 1 mm pool is a fair representation of the absorption rate in a typical tower. Because both the encapsulated liquid sorbent and pool have the same composition, a meaningful comparison of their CO 2 absorption kinetics can be made. To test the kinetics and capacity of the capsules over multiple absorption–regeneration cycles, we used the sealed chamber and pressure measurement described. To regenerate the capsules after each exposure, we heated the capsules to 90 °C in humid air for 10 min. Details regarding the carbonate capacity, thermodynamics and mass transfer modelling can be found in the Supplementary Methods . How to cite this article : Vericella, J. J. et al. Encapsulated liquid sorbents for carbon dioxide capture. Nat. Commun. 6:6124 doi: 10.1038/ncomms7124 (2015).